Giant spin-driven ferroelectric polarization in TbMnO3under high pressure The recent research on multiferroics has provided solid evidence that the breaking of inversion symmetry by spin order can induce ferroelectric polarization P . This type of multiferroics, called spin-driven ferroelectrics, often show a gigantic change in P on application of a magnetic field B . However, their polarization (<~0.1 μC cm −2 ) is much smaller than that in conventional ferroelectrics (typically several to several tens of μC cm −2 ). Here we show that the application of external pressure to a representative spin-driven ferroelectric, TbMnO 3 , causes a flop of P and leads to the highest P (≈1.0 μC cm −2 ) among spin-driven ferroelectrics ever reported. We explain this behaviour in terms of a pressure-induced magnetoelectric phase transition, based on the results of density functional simulations. In the high-pressure phase, the application of B further enhances P over 1.8 μC cm −2 . This value is nearly an order of magnitude larger than those ever reported in spin-driven ferroelectrics. TbMnO 3 , an orthorhombically distorted perovskite manganite ( R MnO 3 where R =trivalent rare-earth) with the Pbnm space group, is one of the most studied spin-driven ferroelectrics [1] , [2] , [3] . In this compound, its ferroelectric polarization P is induced along the c axis by the inversion-symmetry breaking due to a cycloidal spiral spin order [4] ( Fig. 1a ) through the antisymmetric Dzyaloshinskii–Moriya interaction [5] , [6] . Since the interaction originates from relativistic spin–orbit coupling (SOC), the induced P (0.07~0.08 μC cm −2 ) [1] is much smaller than that in conventional displacive ferroelectrics such as BaTiO 3 . The cycloidal spiral spin order in TbMnO 3 is characterized by a propagation vector (0, k ,1) where k ≈0.28 and results from the competition between ferromagnetic (FM) in-plane nearest ( J 1 ) and antiferromagnetic in-plane next-nearest-neighbour ( J 2 ) interactions of Mn moments [7] . This competition and, in turn, the resulting spin-ordered state, are modified by replacing Tb with other rare-earth ions [8] . By substituting smaller ions such as Ho and Y (that is, applying chemical pressure), the Mn–O–Mn bond angles decrease [9] , leading to the enhancement of J 2 / J 1 (ref. 7 ). As a result, the ground state changes into a collinear up-up-down-down (↑↑↓↓) spin structure, the so-called ‘E-type’ antiferromagnetic (E-AFM) structure [10] , shown in Fig. 1b . Both model Hamiltonian [11] and first-principles [12] calculations predicted another type of spin-driven mechanisms for polarization: ferroelectricity in the E-AFM phase is ascribed to nonrelativistic symmetric exchange striction, which causes substantial atomic displacements (orange arrows Fig. 1b ) and induces relatively large P (~6 μC cm −2 ) along the a axis. In fact, P observed experimentally in E-AFM R MnO 3 (for example, ~0.15 μC cm −2 in polycrystalline TmMnO 3 (ref. 13 ), ~0.17 μC cm −2 in polycrystalline LuMnO 3 (ref. 14 ) and ~0.24 μC cm −2 in a single crystal of YMnO 3 (ref. 15 )) is larger than that in spin-spiral TbMnO 3 . However, the P -value appears one order of magnitude smaller than that predicted theoretically [11] , [12] . 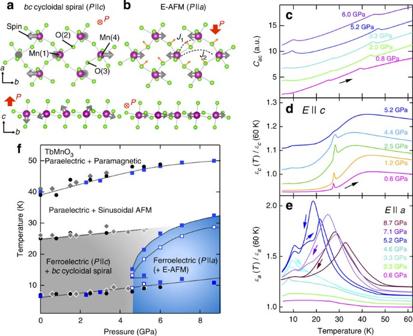Figure 1: Evolution of electric and magnetic phases of TbMnO3by applying pressure. (a,b) Cycloidal spiral (a) and E-AFM (b) structures observed in orthorhombically distorted perovskite manganites. The upper and lower panels show views along thecand theaaxes, respectively. Orange arrows denote directions of atomic displacements due to the symmetric exchange striction at the respective oxygen sites. (c–e) Temperature profiles of heat capacityCac(c) and relative dielectric constant (εc(d) andεa(e)) scaled by the value of 60 K at several pressures. The respective data are vertically offset for clear comparison. The dielectric constant was measured at a.c. electric fields with 10 kHz. (f) Proposed temperature versus pressure phase diagram. The phase boundaries are determined by theTprofiles ofCac(circles),εc(diamonds) andεa(squares) at the respective pressures. Open and closed symbols denote the data points taken on cooling and heating runs, respectively. Figure 1: Evolution of electric and magnetic phases of TbMnO 3 by applying pressure. ( a , b ) Cycloidal spiral ( a ) and E-AFM ( b ) structures observed in orthorhombically distorted perovskite manganites. The upper and lower panels show views along the c and the a axes, respectively. Orange arrows denote directions of atomic displacements due to the symmetric exchange striction at the respective oxygen sites. ( c – e ) Temperature profiles of heat capacity C ac ( c ) and relative dielectric constant ( ε c ( d ) and ε a ( e )) scaled by the value of 60 K at several pressures. The respective data are vertically offset for clear comparison. The dielectric constant was measured at a.c. electric fields with 10 kHz. ( f ) Proposed temperature versus pressure phase diagram. The phase boundaries are determined by the T profiles of C ac (circles), ε c (diamonds) and ε a (squares) at the respective pressures. Open and closed symbols denote the data points taken on cooling and heating runs, respectively. Full size image The application of physical pressure, leading to structural modifications such as shortening of interatomic distance can be another tool to tune the magnetic competition, spin state and resulting spin-driven ferroelectricity [16] . In fact, a powder neutron diffraction study under high pressures on TbMnO 3 indicates that the spiral spin-ordered state transforms into the E-AFM phase at around 3.6 GPa (ref. 17 ). Though there are few works [18] focused on the effects of applied pressure on spin-driven ferroelectricity in TbMnO 3 , these studies have been carried out only up to 1~2 GPa and have never reported drastic changes in the ground state, (such as a pressure-induced ferroelectric phase transition). In this study, we investigated the effects of high pressure—up to 8.7 GPa—on the ferroelectric properties in TbMnO 3 , and discovered a pressure-induced magnetoelectric phase transition and the largest ferroelectric polarization among known spin-driven ferroelectrics. Pressure versus temperature phase diagram Figures 1c–e show temperature T profiles of heat capacity ( C ac ), relative dielectric constant along the c axis ( ε c ) and along the a axis ( ε a ), respectively, at several pressures. The data of the dielectric constant are normalized by data at 60 K. At 0.8 GPa, the T dependence of C ac exhibits three distinct anomalies at around 40 K, 27 K and 7 K, which correspond to the Néel temperature of Mn moments ( ), the ferroelectric transition temperature ( T C ) and the Néel temperature of Tb moments ), respectively. As the applied pressure increases, all of the three anomalies monotonically shift toward higher temperatures. Above 4~5 GPa, the anomaly at T C almost vanishes (see also the phase diagram displayed in Fig. 1f ). Corresponding to this suppression of the heat capacity anomaly at T C , a distinct peak feature observed at T C in ε c is also suppressed above around 5 GPa (see Fig. 1d ). This suggests that ferroelectricity along the c axis disappears above around 5 GPa. By contrast, the application of pressure above around 4.5 GPa induces a striking peak feature accompanying a thermal hysteresis in the T dependence of ε a , as shown in Fig. 1e . In the 5.2-GPa data, the most enhanced peak feature can be seen at around 20 K, at which the maximum value of ε a reaches around 150. The peak structure in ε a − T curves at high pressure reminds us of a ferroelectric phase transition. 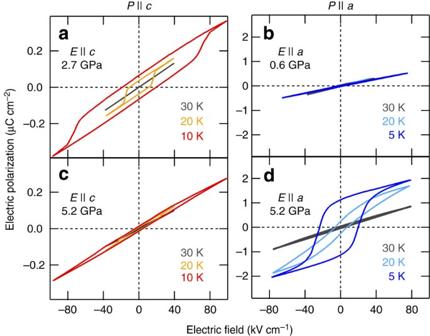Figure 2: Pressure-induced polarization-flop transition of TbMnO3. P–Ecurves measured withEalong thecaxis (a) and theaaxis (b) in the low-pressure phase. Those measured withEalong thecaxis (c) and theaaxis (d) in the high-pressure phase. Pressure effect on P–E curve Figure 2 shows P–E curves collected with applying an electric field ( E ) along the c and a axes at selected pressures. In the data at low pressures ( Fig. 2a,b ), at which a peak feature was observed in ε c − T curves, a clear hysteresis loop was observed only in the P // c configuration. This means that the system is ferroelectric with a spontaneous polarization ( P s ) along the c axis. The P s of 0.07 μC cm −2 and the coercive field of 70 kV cm −1 observed at 10 K and 2.7 GPa ( Fig. 2a ) are nearly the same with those collected at ambient pressure [1] . (The slope of the P–E curves, which is related to the magnitude of the dielectric constant, looks large. This is due to the smallness of P s in the spin spiral. If P s were larger, the slope of P s would be less represented). By contrast, in the data at 5.2 GPa ( Fig. 2c,d ), at which ε a − T curves exhibit a distinct peak structure, no substantial hysteresis loop was observed in the P // c configuration, while that of P//a shows a gigantic hysteresis loop characteristic of ferroelectric along the a axis. The results shown in Figs 1 and 2 demonstrate that TbMnO 3 exhibits a pressure-induced polarization-flop transition, where the ferroelectric polarization vector is switched from pointing along the c to the a axis by the application of pressure at around 4.5 GPa. These experimental results on the pressure dependence of the ferroelectric properties are summarized in the phase diagram shown in Fig. 1f . Figure 2: Pressure-induced polarization-flop transition of TbMnO 3 . P–E curves measured with E along the c axis ( a ) and the a axis ( b ) in the low-pressure phase. Those measured with E along the c axis ( c ) and the a axis ( d ) in the high-pressure phase. Full size image The most remarkable result of the abovementioned pressure effect is a gigantic magnitude of P s observed in the high-pressure P // a phase. More detailed pressure effects on P–E curves in the high-pressure phase are displayed in Fig. 3a . It is evident that T C , P s and the coercive field tend to increase with increasing pressure from 4.6 GPa to 8.7 GPa. At 5 K, P s reaches a maximum (≈1.0 μC cm −2 ) at 5.2 GPa and turns to be suppressed above 5.2 GPa. The observed P s is larger by an order of magnitude than that in the low-pressure P // c phase and exceeds the highest values ever reported in spin-driven ferroelectrics (c.f., 0.29 μC cm −2 in CaMn 7 O 12 (ref. 19 ) and 0.36 μC cm −2 in GdMn 2 O 5 (ref. 20 )). 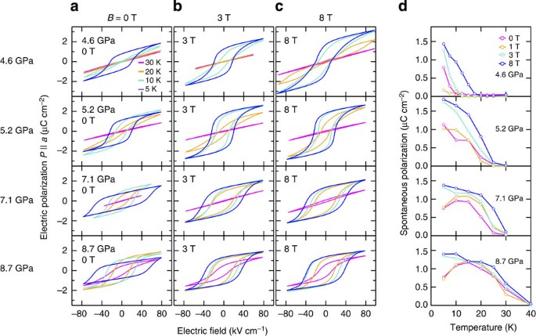Figure 3: Giant spin-driven ferroelectric polarization in the high-pressure phase of TbMnO3. (a–c)P–Ecurves measured withEapplied along theaaxis atB=0 (a), 3 (b) and (c) 8 T. The first, second, third and fourth panels from the top denote the data at 4.6, 5.2, 7.1 and 8.7 GPa. (d) The spontaneous polarizationPsas a function of temperature at various magnetic fields and pressures. Figure 3: Giant spin-driven ferroelectric polarization in the high-pressure phase of TbMnO 3 . ( a – c ) P – E curves measured with E applied along the a axis at B =0 ( a ), 3 ( b ) and ( c ) 8 T. The first, second, third and fourth panels from the top denote the data at 4.6, 5.2, 7.1 and 8.7 GPa. ( d ) The spontaneous polarization P s as a function of temperature at various magnetic fields and pressures. Full size image Density functional theory—pressure-induced phase transition To understand the microscopic origin of the polarization enhancement occurring under pressure, we performed simulations based on first-principles density functional theory (DFT) for different spin configurations (see Methods). 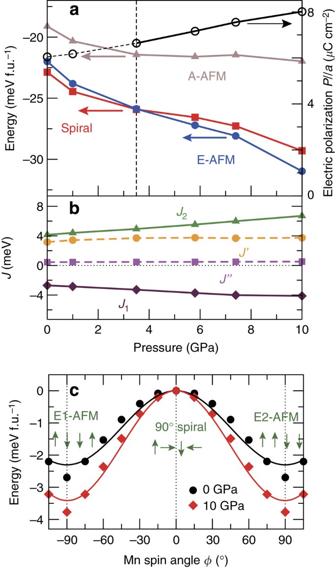Figure 4: Stabilization of the collinear E-AFM phase by applying pressure. (a) DFT-calculated total energy of different magnetic phases with respect to the FM phase, taking into account spin–orbit coupling. Calculated polarization along theaaxis in the E-AFM configuration is also shown. (b) Superexchange energies (Jij): in-plane nearest-neighbour (J1), in-plane next-nearest-neighbour (J2), inter-plane nearest-neighbour (J′) and inter-plane next-nearest-neighbour (J′′). Negative (positive) values favour parallel (antiparallel) spin coupling. (c) Total energy versus orientation of the central Mn spins along an adiabatic polarization-switching path, connecting E1-AFM (P>0,φ=−90°), 90° spiral (P=0,φ=0°), and E2-AFM (P<0,φ=90°) phases. Figure 4a shows the magnetic stability as a function of applied pressure: the cycloid spin structure (with k =1/3) is the magnetic ground state at ambient pressure, whereas the E-AFM becomes the ground state under high pressure (>3.5 GPa). This is consistent with a previous neutron diffraction result on TbMnO 3 (ref. 17 ). In turn, the magnetic transition from the cycloid to the E-AFM phase can qualitatively explain the observed pressure-induced polarization flop transition and the enhancement of P s in the high-pressure phase. The calculated E-AFM-driven ferroelectric polarization along the a axis monotonically increases with increasing pressure ( P s =6.0 μC cm −2 at 0 GPa and P s =8.0 μC cm −2 at 10 GPa (see Supplementary Note 1 )), being two orders of magnitude larger than the spiral-spin-induced polarization at 0 GPa (~0.05 μC cm −2 along the c axis [21] ). This increase is due to the enhancement of Mn- e g electron hopping under pressure (consistent with the bandwidth of occupied e g electronic states increasing from 0.62 to 0.75 eV), related to the so-called ‘asymmetric hopping’ at the basis of the microscopic origin of ferroelectricity [22] . The increase in P s with increasing pressure is inconsistent with the aforementioned experimental results in which P s turns to decrease above 5.2 GPa. One possible explanation for the discrepancy is ascribed to the enhancement of the coercive field with increasing pressure. If that is the case, larger E is needed to fully switch ferroelectric domains, and actual P s at high pressure is larger than that obtained from the data of Fig. 3a . Figure 4: Stabilization of the collinear E-AFM phase by applying pressure. ( a ) DFT-calculated total energy of different magnetic phases with respect to the FM phase, taking into account spin–orbit coupling. Calculated polarization along the a axis in the E-AFM configuration is also shown. ( b ) Superexchange energies ( J ij ): in-plane nearest-neighbour ( J 1 ), in-plane next-nearest-neighbour ( J 2 ), inter-plane nearest-neighbour ( J′ ) and inter-plane next-nearest-neighbour ( J′′) . Negative (positive) values favour parallel (antiparallel) spin coupling. ( c ) Total energy versus orientation of the central Mn spins along an adiabatic polarization-switching path, connecting E1-AFM ( P >0, φ =−90°), 90° spiral ( P =0, φ =0°), and E2-AFM ( P <0, φ =90°) phases. Full size image The stabilization of the E-AFM phase can be understood in terms of the enhancement of both J 1 and J 2 under pressure, with the general trend | J 2 |>| J 1 | (see Fig. 4b ). Our result, J 1 =−2.7 meV and J 2 =4.15 meV at 0 GPa, is consistent with the J -values estimated from neutron scattering [23] , which provides J 1 =−2.4 meV (their reported value J FM =0.15 meV doesn’t include the spin moment S =4 μ B , so J 1 =J FM S 2 should be compared with our results) and the ratio J 2 / J 1 =−0.8. The enhancement of J 1 with increasing pressure can be reasonably explained by the increase of Mn–O–Mn bond angles (145.0° at 0 GPa and 145.8° at 10 GPa in the optimized cell), while that of J 2 is related to structural changes in Mn(1)–O(2)–O(3)–Mn(4) (longer-ranged) interaction paths (see Fig. 1a and Supplementary Note 2 ). In the optimized cell, the O(2)–O(3) bond length d 23 is shortened by pressure (3.075 Å at 0 GPa to 3.040 Å at 10 GPa), as shown in Supplementary Fig. 1 . As a result, under pressure the strongly enhanced J 2 (antiparallel spin coupling) and slightly weaker J 1 (parallel spin coupling) stabilize the ↑↑↓↓ E-AFM spin configuration. In R MnO 3 , it is well known that the lattice contraction by chemical pressure, that is, substitution of R site with smaller rare-earth, mainly causes the decrease of the Mn–O–Mn bond angles [9] . In contrast, the application of physical pressure shortens Mn–O bond lengths but increases the Mn–O–Mn bond angles [24] , so that both J 1 and J 2 are enhanced, therefore making the E-AFM spin configuration unusually stable in TbMnO 3 under pressure. Since the enhancement of J 1 and J 2 is simply ascribed to the enhancement of the Mn- e g electron hopping between the nearest-neighbour and the next-nearest-neighbour Mn sites, it is fair to say that the characteristic lattice deformation caused by applying pressure leads to large ferroelectric polarization in the high-pressure phase. In this context, high pressure is needed to obtain larger ferroelectric polarization from E-AFM R MnO 3 . However, we don’t deny the possibility that such lattice deformation is realized at ambient pressure by special synthesis techniques such as high-pressure synthesis and epitaxial thin-film growth. Effect of biquadratic spin–phonon interaction Another ingredient favouring the collinear E-AFM configuration is the biquadratic spin–phonon interaction (see Methods). As shown in Fig. 4c , we simultaneously rotated half of the Mn spins from ↑→↓← (90° spiral) to ↑↑↓↓ E-AFM configuration [25] . Along this spin rotation path, the exchange interaction J ij ( S i ˙ S j ) doesn’t contribute to the energy lowering, the latter being then exclusively due to the spin–phonon interaction − B biq ( S i ˙ S j ) [2] (refs 26 , 27 ). Indeed, B biq is also enhanced from 2.2 meV f.u. −1 (at 0 GPa) to 3.2 meV f.u. −1 (at 10 GPa), therefore contributing to the stabilization of the collinear E-AFM phase under pressure. Both the preference for the E-AFM configuration and the polar ionic distortion originate from the same root, namely, the asymmetric hopping mechanism. Under pressure, the enhanced e g electron hopping also increases spin–phonon interaction. By aligning the spins in the ↑↑↓↓ configuration, a spin-Peierls-like mechanism makes Mn ions to dimerize, in order to increase hopping between the same spin sites and decrease hopping between opposite spin sites, therefore reducing the kinetic energy. At the same time, exchange striction becomes active in the symmetry-lowered spin configuration, which displaces O ions between Mn ions in the polar distortion mode. This plays a key role in the lattice-induced contribution to polarization in E-AFM. Effect of magnetic fields on ferroelectricity under high pressure Next we investigated the effect of a magnetic field B applied along a on the giant spin-driven P in the high-pressure P//a phase. In Fig. 3a–c , we plot P–E curves measured at various T , B and pressures above 4.6 GPa. These P − E hysteresis loops clearly show that the ferroelectric polarization in the high-pressure P // a phase is strongly affected by B . From these data, the T profiles of P s at the respective B and pressures are summarized in Fig. 3d , in which one can find that the maximum of P s reaches 1.8 μC cm −2 at 5 K, 8 T and 5.2 GPa. This value for a spin-driven ferroelectric is nearly of the same order of magnitude as that of conventional ferroelectrics (for example, ~4 μC cm −2 in triglycine sulphate, (NH 2 CH 2 COOH) 3 ·H 2 SO 4 (ref. 28 ) and ~20 μC cm −2 in barium titanate, BaTiO 3 (ref. 29 )). To further elucidate the B effect on P in the high-pressure phase, we investigated magnetodielectric and magnetoelectric effects at 7.1 GPa. 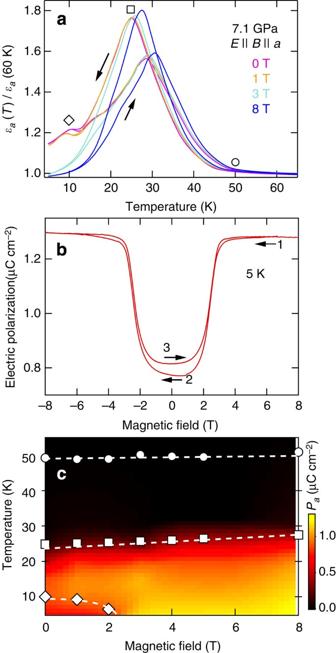Figure 5: Giant magnetoelectric effect observed in the high-pressure phase of TbMnO3. (a) Temperature profiles ofεascaled by the value of 60 K at 7.1 GPa and several magnetic fields. (b) Magnetic-field-induced change in electric polarization at 5 K and 7.1 GPa. (c) Temperature versus magnetic-field phase diagram superimposed on the contour map of the value of induced electric polarization at 7.1 GPa. Open circles, squares and diamonds denote the temperature at whichεa–Tcurves exhibit a steep increase ofεatoward lowT, a peak structure and a small shoulder, respectively. Here we adopt the data taken on cooling. BothEandBare applied along theaaxis. Figure 5a displays ε a − T curves at 7.1 GPa in the presence of selected magnetic fields. These ε a − T curves with a distinct thermal hysteresis can be characterized by three anomalies: a steep increase of ε a toward low T at 45~50 K (indicated by open circle), a peak structure at 25~30 K (open square) and a small shoulder at around 10 K (open diamond). Taking account of the results at ambient pressure [1] , these anomalies probably represent magnetic (and ferroelectric) transition points. The peak structure related to the ferroelectric transition slightly shifts toward higher T with increasing B . It should be also noted that the small shoulder disappears by applying B above 2~3 T and the magnitude of ε a at the lowest T is considerably suppressed. Figure 5b displays a direct magnetoelectric effect, that is, a change in P by sweeping B , at 5 K and 7.1 GPa. At around | B |=2~3 T, the magnitude of P increases rapidly from 0.8 to 1.3 μCcm −2 . As shown in Fig. 5b , the B -induced change in P persists in both B -increasing and B -decreasing runs, and reaches 0.5 μC cm −2 which is comparable with the highest value ever observed in spin-driven ferroelectrics (for example, 0.5 μC cm −2 in GdMn 2 O 5 (ref. 20 )). Figure 5: Giant magnetoelectric effect observed in the high-pressure phase of TbMnO 3 . ( a ) Temperature profiles of ε a scaled by the value of 60 K at 7.1 GPa and several magnetic fields. ( b ) Magnetic-field-induced change in electric polarization at 5 K and 7.1 GPa. ( c ) Temperature versus magnetic-field phase diagram superimposed on the contour map of the value of induced electric polarization at 7.1 GPa. Open circles, squares and diamonds denote the temperature at which ε a –T curves exhibit a steep increase of ε a toward low T , a peak structure and a small shoulder, respectively. Here we adopt the data taken on cooling. Both E and B are applied along the a axis. Full size image The magnetoelectric effect observed in the high-pressure P//a phase is arranged in Fig. 5c as a T versus B phase diagram stacked with the contour plot of the magnitude of P . As seen in the phase diagram, there are two distinct ferroelectric phases with different magnitude of ferroelectric polarization (separated by the phase boundary marked by diamond symbols). At the lowest T , P is steeply enhanced by applying B above ~2 T. In the case of the ambient-pressure condition, it is known that the application of B along the a axis causes a flop of P from the P//c phase with the bc cycloid to the P//a phase with the ab cycloid [30] , [31] . That is, the application of B along a stabilizes the P//a phase at ambient pressure. In terms of the stabilization of P//a state, the high-pressure phase exhibits a similar tendency. The P flop observed at ambient pressure is interpreted as a result of reduced Tb–Mn exchange interaction when Tb moments become aligned ferromagnetically by applying B [32] . Because of a lack of information about magnetism in the high- B phase under high pressure, we cannot confirm the origin of the presently observed enhancement of P above ~2 T at this stage. However, taking account of the results at ambient pressure, it is natural to speculate that B -induced change in the ordered state of Tb moments contributes to the observed enhancement of P by applying B through the Tb–Mn symmetric exchange striction. However, to clarify the origin of the B -enhanced P observed in the high-pressure phase in more detail, we will need more information about magnetic properties which can be obtained from in-field magnetization and neutron-scattering measurements under high pressure. Though the detailed mechanism is still an open question, the drastic change in P by applying B confirms that the observed gigantic ferroelectric polarization is ascribed to a spin-driven origin. To conclude, we carried out dielectric measurements on TbMnO 3 under high pressure, and found the pressure-induced magnetoelectric phase transition and the largest ferroelectric polarization among spin-driven ferroelectrics ever reported. These results were qualitatively explained by the density functional simulations. Our study demonstrated that it is possible to attain gigantic spin-driven ferroelectric polarization which is nearly of the same order of magnitude as that in conventional ferroelectrics, and to control it magnetically. Another aspect for the present finding is that the application of high pressure can be an effective perturbation to achieve high-performance multiferroics. Experimental procedure A single crystal of TbMnO 3 was grown by the floating zone method. The crystal was cut into thin plates (typical dimensions, ≈150 × 150 × 25 μm 3 ) with the widest surfaces perpendicular to the a or c axis (in the Pbnm notation). Heat capacity obtained by ac -calorimetry ( C ac ), relative dielectric constant ( ε ) and electric polarization ( P ) were measured at various pressures by using a diamond anvil cell (DAC) made of Cu–Be alloy. For the measurements of ε and P , an electric field ( E ) was applied along the a or c axis. Glycerine was used as a pressure-transmitting medium, which remains liquid up to around 5 GPa at room temperature. Pressure was applied at room temperature and determined at room temperature and 10 K for the respective measurements by the ruby fluorescence method. The DAC was introduced into a superconducting magnet which allows the control of temperature ( T ) and the application of a magnetic field ( B ). A lock-in amplifier and an LCR meter (L: inductance, C: capacitance, R: resistance) were used for the measurements of C ac and ε , respectively. More details of the experimental techniques have been reported in refs 33 and 34 . To obtain the E ( B ) dependence of P , displacement current was measured with an electrometer while sweeping E at a rate of 60 kV cm −1 min −1 (sweeping B at a rate of 1 T min −1 ). These current measurements were performed after poling the crystals at 70~100 kV cm −1 while cooling from 60 K to measurement temperature. By integrating the displacement current as a function of time, P was obtained. All the P data shown in this paper were taken during the cooling procedure. Measurements of ε and P in applied B were done in the configuration with B parallel to E . Density functional simulations Density functional simulations were performed using the Vienna Ab Initio Simulation Package [35] , within the generalized gradient approximation [36] to the exchange correlation potential. We note that the use of GGA+ U potential worsens the results, leading to an A-type antiferromagnetic (A-AFM) ground state in the whole pressure range (the worse DFT+ U results for manganites have been discussed at length in ref. 25 ). We followed a procedure similar to ref. 22 . First, we optimized internal atomic parameters imposing the A-AFM spin configuration, whereas we took the experimental lattice parameters under pressure from ref. 24 (note that measurements have been done at room temperature). We also extracted additional sets of lattice parameters by linearly interpolating experimental values. By using this optimized cell, we compared total energies of several magnetic configurations, that is, A-, C-, G-, E-, E*-AFM in a × 2 b × c orthorhombic Pbnm supercell and cycloidal-spin structure (with k =1/3 spiral in the bc plane) in a × 3 b × c supercell, with reference to FM in respective supercells. Here, A-, C-, G- and E-AFM denote spin configurations in the standard Wollan–Koehler notation [37] , while E*-AFM represents the spin configuration showing the same in-plane spin arrangement as E-AFM but with an interplanar FM coupling [22] . The cutoff energy for plane waves was set at 500 eV, whereas the k -point sampling was done using the 4 × 2 × 3 and 4 × 1 × 3 Monkhorst-Pack k -point grid, respectively. The numerical error caused by using a different size for the supercells was evaluated by comparing energy differences between A-AFM and FM, calculated in the two supercells: the numerical error was less than 2 meV f.u. −1 . As a second step, in order to discuss ferroelectric properties, the internal atomic structure was further optimized within the E-AFM spin configuration, leading to ferroelectric polarization induced by exchange striction, as discussed in E-AFM HoMnO 3 (ref. 12 ). We note that SOC doesn’t significantly change the magnetic stability. Ferroelectric polarization was calculated by using the Berry phase method. The calculated magnetic energy was mapped to the following Hamiltonian, The first term is the conventional Heisenberg exchange term, while the second term represents the biquadratic spin interaction related to spin–phonon coupling; the latter tends to favour a collinear spin alignment, therefore stabilizing the E-AFM order with respect to cycloidal orders [26] , [38] . In the Hamiltonian, the spin moment was normalized to 1. In order to disentangle the role of SOC, we performed DFT simulations with and without SOC; since the energy ordering of different phases did not change and the whole-phase diagram was only marginally affected, in our Hamiltonian we neglected any term related to SOC (such as single-ion anisotropy, Dzyaloshinskii–Moriya terms and so on). How to cite this article: Aoyama, T. et al. Giant spin-driven ferroelectric polarization in TbMnO 3 under high pressure. Nat. Commun. 5:4927 doi: 10.1038/ncomms5927 (2014).